No-go theorem for superradiant quantum phase transitions in cavity QED and counter-example in circuit QED In cavity quantum electrodynamics (QED), the interaction between an atomic transition and the cavity field is measured by the vacuum Rabi frequency Ω 0 . The analogous term 'circuit QED' has been introduced for Josephson junctions, because superconducting circuits behave as artificial atoms coupled to the bosonic field of a resonator. In the regime with Ω 0 comparable with the two-level transition frequency, 'superradiant' quantum phase transitions for the cavity vacuum have been predicted, for example, within the Dicke model. In this study, we prove that if the time-independent light-matter Hamiltonian is considered, a superradiant quantum critical point is forbidden for electric dipole atomic transitions because of the oscillator strength sum rule. In circuit QED, the analogous of the electric dipole coupling is the capacitive coupling, and such no-go property can be circumvented by Cooper pair boxes capacitively coupled to a resonator, because of their peculiar Hilbert space topology and a violation of the corresponding sum rule. Cavity [1] and circuit [2] quantum electrodynamics (QED) are fascinating topics because of the ultimate manipulation of light-matter interaction at the quantum level. In particular, the remarkable control of two-level systems and their coupling to the quantum field of a resonator can pave the way for the realization and study of new quantum phases for fundamental studies and quantum applications. The physics of a system consisting of N atoms coupled to the same quantum field of a photonic mode has generated tremendous interest since the celebrated paper by Dicke [3] on atomic superradiance. The Dicke model Hamiltonian is equivalent to a collection of 1/2-pseudospins (two-level systems) coupled to the same bosonic field. In the past, it was suggested that such a system can undergo a classical phase transition [4] , that is, occurring at a finite temperature. Remarkably, in such a phase transition, the system exhibits a spontaneous polarization of the atoms and a spontaneous coherent electromagnetic field. The Dicke model Hamiltonian also exhibits a quantum phase transition [5] , which can occur at zero temperature by tuning the light-matter coupling across a quantum critical point [6] . Above the quantum critical point, the vacuum (ground state) of the cavity system is twice degenerate. A linear superposition of these two degenerate ground states can be seen as a collective qubit characterized by a strong light-matter entanglement (the cavity field is in a coherent state, the matter part in a 'ferromagnetic' phase). In the case of the classical phase transition for the Dicke model, such a prediction was challenged by a no-go theorem [7] , [8] , [9] . In fact, the Dicke Hamiltonian is obtained by neglecting the squared electromagnetic vector potential Â 2 in the light-matter quantum Hamiltonian, but it was shown that by including such a fundamental term in the Dicke Hamiltonian, the finite-temperature classical phase transition disappears in the case of electric dipole coupling [7] , [8] , [9] , [10] . Note that recent works in atomic cavity QED [11] , [12] have followed a dynamic approach to achieve a Dicke-like transition, that is, by using time-dependent applied fields dressing the system. However, to have a genuine quantum phase transition and stable quantum phases associated to collective eigenstates, it is an important and fundamental matter to explore original approaches based on time-independent Hamiltonians in circuit QED. Indeed, a fundamental and general problem to be investigated is whether intrinsic limitations occurring for cavity QED systems can translate necessarily into analogous constraints for superconducting circuit QED systems. In this paper, we show that in the case of cavity QED systems consisting of real atoms (coupled through their electric dipole), the due inclusion of the Â 2 -term in the Dicke Hamiltonian forbids the quantum phase transition as a consequence of the Thomas-Reiche-Kuhn (TRK) sum rule for the oscillator strength. Note that our proof is obtained by considering the time-independent quantum light-matter Hamiltonian. Remarkably, we show that such no-go property does not necessarily hold for the analogous circuit QED system, namely, a collection of Josephson atoms capacitively coupled to a transmission line resonator (see Fig. 1 ). We show that by taking as artificial atoms a collection of Cooper pair boxes, the corresponding quantum Hamiltonian has the same form as the cavity QED counterpart, but, importantly, it has different constraints between the coupling constants. The peculiar topology of the Cooper pair box wavefunction is shown to be essential for the violation of the corresponding sum rule and the appearance of a quantum critical point in the case of capacitive coupling. Our work shows that superconducting quantum circuits [13] are not only appealing for the remarkable strength of the light-matter interaction but they also can give rise to artificial atoms with qualitatively different behaviour when compared with real atoms. 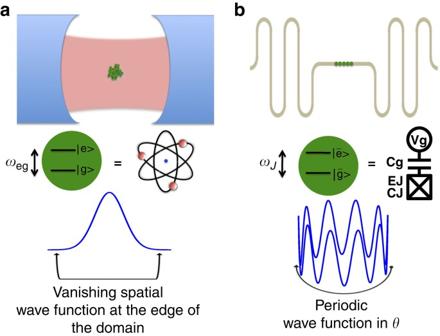Figure 1: Sketch of the two considered systems. (a) Collection ofNidentical atoms coupled by their electric dipole to the quantum field of a cavity resonator. (b) Collection ofNCooper pair boxes capacitively coupled to a transmission line resonator. Figure 1: Sketch of the two considered systems. ( a ) Collection of N identical atoms coupled by their electric dipole to the quantum field of a cavity resonator. ( b ) Collection of N Cooper pair boxes capacitively coupled to a transmission line resonator. Full size image The case of cavity QED Let us consider a collection of N identical and isolated atoms that do not interact directly with each other (see Fig. 1 ). This is equivalent to considering the Hamiltonian: where H j is the bare Hamiltonian for the j -th atom, i j denotes one of the ν particles of charge q i constituting the atom; is the corresponding momentum (mass) entering the non-relativistic kinetic energy, whereas U j is the generic potential energy depending on the position coordinates. Of course, for atoms made of electrons we have and q i j = − e , but what follows is valid for the general case of different masses and charges. To account for the interaction of the atoms with the quantum field in the cavity resonator, we have to perform the standard minimal coupling replacement, namely, . If we consider only one resonant photonic mode and hypothesize that in the region occupied by the atoms the spatial variation of the field is negligible, we can replace Â ( r ) with A 0 ( a † + a ), where a † ( a ) is the corresponding bosonic photon creation (annihilation) operator and A 0 is the vector potential field in the region occupied by the atoms. Therefore, we obtain the interaction term as well as the A 2 term If we consider each atom as a two-level system (|g› and |e› are the two eigenstates for each atom) and if we use the fundamental commutation relation we get: with ω eg = ω e − ω g , the atomic transition frequency, and where the electric dipole matrix element is It is convenient to introduce the bright excitation operators (bosonic in the 'thermodynamical' limit N 1): in order to express the interaction Hamiltonian in the form: where is the collective vacuum Rabi frequency accounting for the -enhancement of the coupling. The Â 2 term instead takes the form Finally, the atomic part of the Hamiltonian can be written as where we have omitted the bare energy of the dark excitations (the matter collective excitation modes not coupled to the cavity mode and orthogonal to the bright mode). Considering only one photonic mode, the cavity energy reads By using an Hopfield–Bogoliubov transformation [14] , [15] , it is possible to rewrite the Hamiltonian in the form: where the collective bosonic modes operators P + and P − satisfy and Such operators are defined as where the coefficient vectors are eigenvectors of the Hopfield–Bogoliubov matrix M : The corresponding positive eigenvalues directly give the frequencies ω + and ω − of the two collective modes. In this formalism, a quantum critical point is obtained when the determinant of M vanishes, because one excitation becomes gapless (zero eigenvalue). Such a determinant is simply given by Note that by using a Holstein–Primakoff approach [16] , [17] (details not shown), one finds the same equation Det ( M )=0 for the quantum critical point. In the case of the Dicke Hamiltonian, the Â 2 term is neglected; hence D =0 and the condition Det ( M )=0 gives the quantum critical coupling Above a critical coupling, a symmetry breaking occurs, the ground state (vacuum) becomes twice degenerate, a spontaneous coherence for light and matter fields appears (the bosonic excitations have to be considered around the symmetry breaking vacua, for example, by a Holstein–Primakoff approach [16] , [17] ). 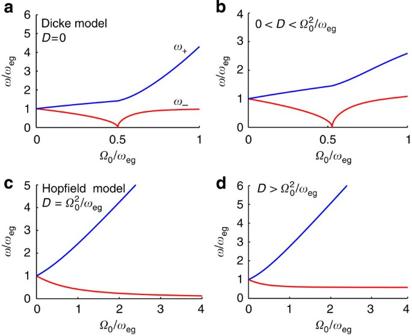Figure 2: Normalized frequencies of the two collective bosonic excitation branches. We have derived the bosonic collective excitation frequenciesω+(blue line) andω−(red line) as a function of the normalized vacuum Rabi frequency. We have considered the case of an atomic transition frequency equal to the cavity frequency. For the two considered systems (seeFig.1), the form of the quantum Hamiltonian is identical and depends on four physical quantities: the resonator mode frequency; the two-level transition frequencyωeg; the collective vacuum Rabi frequency Ω0; the amplitude frequencyDof the Hamiltonian term quadratic in the resonator boson field. In the case of cavity QED, this term is due to the squared electromagnetic vector potential. In the considered class of circuit QED systems (Cooper pair boxes capacitively coupled to a resonator), it comes from the squared voltage field operator. The frequenciesω+andω−are very sensitive to the relation between Ω0andD, with four possible cases: (a)D=0 (no term quadratic in the resonator quantum field). It corresponds to the Dicke model. A quantum critical point (with a gapless excitation frequency) occurs for Ω0/ωeg=0.5 (the energies above this point are calculated using a Holstein–Primakoff approach16,17). According to our proof, this limit cannot be obtained in cavity QED with atoms coupled through the electric dipole (without time-dependent applied fields). (b)In this case, the superradiant quantum phase transition is still possible, but with a shifted quantum critical point. This case is still not accessible to the considered cavity QED system, but it can be achieved with Cooper pair boxes in circuit QED. In the simulation,(it can be obtained with circuit parameters such thatEJ/(4Ec)=0.1). (c)The quantum critical point disappears andω−→0 for Ω0→+∞. This corresponds to the Hopfield model15. It can be obtained in cavity QED if the electric dipole transition takes all the oscillator strength. (d)The frequencyω−is finite even in the ultrastrong coupling limit. In Figure 2a , excitation frequencies are shown for the Dicke case D =0 (taking ω cav = ω eg ). The ω − branch vanishes at the quantum critical point. However, if the Â 2 term is retained, the situation changes dramatically. In fact, by using the Cauchy-Schwartz inequality, we get Figure 2: Normalized frequencies of the two collective bosonic excitation branches. We have derived the bosonic collective excitation frequencies ω + (blue line) and ω − (red line) as a function of the normalized vacuum Rabi frequency. We have considered the case of an atomic transition frequency equal to the cavity frequency. For the two considered systems (see Fig.1 ), the form of the quantum Hamiltonian is identical and depends on four physical quantities: the resonator mode frequency; the two-level transition frequency ω eg ; the collective vacuum Rabi frequency Ω 0 ; the amplitude frequency D of the Hamiltonian term quadratic in the resonator boson field. In the case of cavity QED, this term is due to the squared electromagnetic vector potential. In the considered class of circuit QED systems (Cooper pair boxes capacitively coupled to a resonator), it comes from the squared voltage field operator. The frequencies ω + and ω − are very sensitive to the relation between Ω 0 and D , with four possible cases: ( a ) D =0 (no term quadratic in the resonator quantum field). It corresponds to the Dicke model. A quantum critical point (with a gapless excitation frequency) occurs for Ω 0 / ω eg =0.5 (the energies above this point are calculated using a Holstein–Primakoff approach [16] , [17] ). According to our proof, this limit cannot be obtained in cavity QED with atoms coupled through the electric dipole (without time-dependent applied fields). ( b ) In this case, the superradiant quantum phase transition is still possible, but with a shifted quantum critical point. This case is still not accessible to the considered cavity QED system, but it can be achieved with Cooper pair boxes in circuit QED. In the simulation, (it can be obtained with circuit parameters such that E J /(4 E c )=0.1). ( c ) The quantum critical point disappears and ω − →0 for Ω 0 →+∞. This corresponds to the Hopfield model [15] . It can be obtained in cavity QED if the electric dipole transition takes all the oscillator strength. ( d ) The frequency ω − is finite even in the ultrastrong coupling limit. Full size image By using the TRK sum rule for the electric dipole oscillator strength (for details see Methods), we get The general inequality implies that Det ( M ) never vanishes (as it can be verified in a straightforward manner by inspecting the expression in Equation (11)) and that the quantum critical point does not exist any longer (see Fig. 2c and d ). It is interesting to note that the last inequality also prevents a classical superradiant phase transition [7] , [9] . In conclusion, under rather general hypothesis, we have proved that the quantum critical point disappears in the presence of the Â 2 term. The reason is that, as shown by Equation (13), the amplitude of the Â 2 term is not independent of the vacuum Rabi coupling. On the contrary, the Â 2 term becomes even dominant in the ultrastrong coupling regime (Ω 0 / ω eg ≫ 1 implies D ≫ Ω 0 ). We point out that such no-go proof does not concern the case of magnetic coupling (that is, with an interaction Hamiltonian between real spins and a quantized magnetic field [10] ), but is valid in the case of electric dipole transitions and if no external optical fields are applied to the system. The case of circuit QED Here, we show why the fundamental limitation for the superradiant quantum phase transitions, which we have proved under rather general assumptions for the case of cavity QED based on electrical dipole coupling, does not generally apply to superconducting circuit QED. In the case of superconducting Josephson atoms, and (phase and number operator, respectively) have a role analogous to electron spatial position and momentum operators for a real atom. When a Josephson junction is embedded in a transmission line resonator, its degrees of freedom are coupled to the bosonic quantum field of the resonator. In circuit QED, there are many types of artificial atoms depending on the connection of the Josephson junctions to capacitors and inductors. The analogous of the electric dipole coupling is given by the so-called capacitive coupling, whereas the magnetic coupling in cavity QED corresponds to the inductive coupling [18] , [19] . The quantum phase transitions of a chain of inductively coupled Josephson atoms were recently investigated in the study by Nataf and Ciuti [19] . In this article, we will treat the important case of capacitive coupling in circuit QED. As an artificial atom, we will consider a Cooper pair box and show that the peculiar wavefunction topology of such a system can lead to the appearance of a superradiant quantum critical point because of a violation of the sum rule. Therefore, let us consider a chain of Cooper pair boxes embedded in a transmission line resonator [20] . For simplicity, we consider that the Josephson atoms are placed in the middle of the resonator in a small region where the spatial variation of the resonator field is negligible. Moreover, we consider only one resonator mode. With these assumptions (analogous to what was carried out in the case of cavity QED for real atoms), the resonator quantum voltage is where α and α † define the bosonic annihilation and creation operators of the resonator field. The quantum Hamiltonian then reads with the charging energy, E J the tunable Josephson energy. Finally, is the excess charge in the j -th Cooper pair box depending on the static control gate voltage ( V g ) j and the quantum voltage . Here, we will consider the ideal situation of identical Cooper pair boxes such as In each artificial atom, the two-level subspace is obtained by keeping only the two first number states | n =0> and | n =1>. In such a subspace, for n g =1/2, the eigenstates of a Cooper pair box due to the Josephson coupling are and whereas the transition energy is As it is clear that ( − n g ) is analogous to the electron momentum, ( − n g ) is analogous to the p . Â coupling term, whereas 2 is reminiscent of the Â 2 term. The interaction between the resonator quantum field and the charge of the Cooper pair boxes reads as follows: which is analogous to the interaction term in Equation (4). The Hamiltonian contribution due to the 2 term reads as follows: As in the case of cavity QED, we introduce the operator and we have with The sum of the bare energies of the Cooper pair boxes reads (as in the case of real atoms, we have omitted the dark matter excitations, orthogonal to the bright mode and uncoupled to the resonator mode). To determine the excitation bosonic modes of the total quadratic Hamiltonian one can use the Hopfield–Bogoliubov transformation for which one has to diagonalize the matrix By looking at the matrix in Equation (10), it is clear that in the considered circuit QED system, we have found a Hamiltonian of the same form as the one obtained for the cavity QED case. However, there is a fundamental difference, which is crucial for the existence of a superradiant quantum critical point: the relation between the vacuum Rabi frequency 0 and the term originating from the square of the resonator field. In fact, we have Hence, in contrast to the cavity QED case, can be made smaller than In particular, then In such a case, the quantum critical point is shifted by the finite term, but it still exists (see Fig. 2b ). Indeed, the equation det( ) = 0 gives the quantum critical coupling: Note that the limit is also the one in which the two-level approximation for the Cooper pair box is excellent. What is the difference with respect to the cavity QED atomic case? The key issue here is that the wavefunction of a Cooper pair box has a different topology when compared with the wavefunction of a real atom. In the case of a real atom, the wavefunction is not periodic. The commutator between position and momentum is proportional to the identity operator, namely, [ x , p x ] = iħ . Instead, in the case of a Cooper pair box, the charge is quantized and correspondingly the wavefunction is periodic with respect to the phase θ , the phase difference across the junction. In the phase representation, the Cooper pair box wavefunction is such that In other words, there is a circular topology that changes the algebraic rules of the Hilbert space where the physical states 'live'. In particular, the commutator between the phase operator (analogous to the position) and the number operator (analogous to the momentum) is not always proportional to the identity operator. This is crucial because the TRK sum rule for the atomic oscillator strength comes from the fact that [ x , p x ] is proportional to the identity. Indeed, the TRK sum rule is responsible for the inequality in the case of real atoms. In the case of Cooper pair boxes, we have indeed shown that, by choosing a large capacitance energy E c , it is possible to strongly violate the sum rule and therefore allow the existence of a quantum critical point. Note that the violation of the TRK sum rule has been already studied in the context of quantum rigid rotators [21] , which have a different topology with respect to real atoms, but are similar to the Cooper pair box. Here, the fundamental topological properties of the Cooper pair box have very important consequences on the collective behaviour of the chain in a resonator and on the existence of a quantum critical point for the case of capacitive coupling. In the considered circuit QED systems, the corresponding quantum Hamiltonians are time independent (no applied pump fields dressing the system). The predicted quantum phase transition occurs at zero temperature and affects the quantum ground state (vacuum) subspace. Above the quantum critical point, there are two degenerate eigenstates where |α> is a coherent state for the cavity mode and In principle, one could encode quantum information in linear superpositions of such collective vacua, which have been shown to enjoy some protection with respect to local noise sources [19] . It is important to point out that, in atomic cavity QED systems, interesting dynamical approaches to achieve a superradiant transition have been proposed [11] using applied laser fields, and a recent impressive experimental demonstration has been reported [12] (using a coherently dressed Bose–Einstein condensate). In the dynamical case, observables can indeed show interesting discontinuities and symmetry breaking signatures around the critical coupling. However, with respect to the time-independent case, in the dynamic configuration, the system continuously emits (Raman) photons. In fact, in a dynamical approach with time-dependent pump fields, one can obtain a Dicke Hamiltonian only in the pump rotating frame (equivalently, in the case of applied time-dependent fields dressing a three-level system, an Hopfield-like Hamiltonian with the inclusion of A 2 term has also been shown to be obtained in the rotating frame only [22] ). As clearly proven in the general paper by Brown [23] , in such a rotating frame, the Hamiltonian describing the coupling of the system to the environment (for example, the extracavity electromagnetic field) becomes time dependent and has an impact on the coherence properties. Namely, in the case of an open system with dressing time-dependent fields, the Hamiltonian H syst ( t ) does depend on time. If the dressing fields are monochromatic (for example, a pump field with a time dependance as e - i ω p t ), one can conveniently pass to the so-called rotating frame to eliminate such time dependence. In such a frame, the Hamiltonian becomes where U ( t ) is the unitary transformation connecting the laboratory frame to the rotating frame. In the rotating frame, the Hamiltonian syst does not depend on time and one can define pseudo-eigenstates, such that In a dynamical approach for the superradiant transition, syst is the Dicke Hamiltonian. However, the Hamiltonian term describing the interaction with the reservoir becomes time dependent. Namely, one finds Therefore, if one prepares the system in the rotating frame Dicke pseudo-ground state such a state will not be stationary. In particular, the reservoir Hamiltonian syst–bath ( t ) can induce transitions from the pseudo-ground state to excited pseudo-eigenstates, even if the reservoir is at zero temperature. In the laboratory frame, this corresponds to the continuous emission of photons by the system. Consequently, the steady state of the open system in the dynamical configuration is not a pure eigenstate of the Dicke Hamiltonian syst , but a more complex non-equilibrium state. In particular, it is not possible to have stable superpositions between the two degenerate ground states of the Dicke Hamiltonian. Hence, we believe that circuit QED systems with time-independent Hamiltonians have a considerable interest in this respect. In conclusion, we have proven that, under rather general assumptions (electric dipole coupling, two-level atoms, single-mode resonator field), for the case of real atoms in a cavity, the superradiant Dicke quantum phase transition disappears if the Â 2 term is correctly included in the quantum light-matter Hamiltonian. We have shown that the oscillator strength sum rule is what forbids the existence of a quantum critical point. For comparison, we have considered the circuit QED system consisting of a collection of Josephson atoms capacitively coupled to a transmission line resonator, being the capacitive coupling in circuit QED the analogous of electric dipole coupling in cavity QED. We have shown that it is possible to obtain the same quantum Hamiltonian as for the cavity QED case. However, by considering a Cooper pair box as an artificial Josephson atom, we have shown that it is possible to have a quantum critical point. The peculiar circular topology of the Cooper pair box wavefunction prevents the same fundamental limitation imposed by the oscillator strength rule. Our theoretical work shows that circuit QED can provide access to interesting physical effects, which are not necessarily obtained in the analogous cavity QED system, in spite of formal analogies. These original properties may pave the way to exciting avenues towards the realization of interesting quantum phases for fundamental studies and quantum applications. The TRK sum rule Here, we show in detail why the TRK sum rule leads to the inequality in Equation (13). Let us call | g > j and | e > j as the two eigenstates of the j -th atom. Using the fundamental commutation relation we have for where we introduced the dipole operator As all the atoms are identical, we can omit the index j to simplify the notations: We then define d eg =‹e|d|g›=| d eg | u with u as a unitary vector. In the last derivation, on purpose we made explicit two integrals the difference of which results in zero with the sufficient condition of vanishing wavefunctions (and their first and second derivatives) at the edge of the quantization box volume V , as we can see after a double integration by parts. Such boundary conditions are of course valid in the case of atomic states, as their spatial wavefunctions and all their derivatives vanish at the infinity. This is not valid in general for Cooper pair boxes, in which eigenstates have wavefunctions 2π-periodical in θ , the phase difference across the junction. Indeed, the Cooper pair box eigenstates are linear superpositions of quantized charge states {| n >} n ∈ Z in which wavefunctions are Now, to get the inequality (13), we write Using the completeness relation denoting the generic atomic eigenstate, and using we get: where the quantity is proportional to the oscillator strength of the atomic transition between | g > and |σ> in the direction u . If this oscillator strength sum rule is applied to Equation (12), one finally obtains the inequality (13). For the Cooper pair box, because of the circular topology of the wavefunction, the commutator between charge and phase operator is not always proportional to the identity and the sum rule does not hold. How to cite this article : Nataf, P. and Ciuti, C. No-go theorem for superradiant quantum phase transitions in cavity QED and counter-example in circuit QED. Nat. Commun. 1:72 doi: 10.1038/ncomms1069 (2010)